Loss of IP3R-dependent Ca2+signalling in thymocytes leads to aberrant development and acute lymphoblastic leukemia Calcium ions (Ca 2+ ) function as universal second messengers in eukaryotic cells, including immune cells. Ca 2+ is crucial for peripheral T-lymphocyte activation and effector functions, and influences thymocyte selection and motility in the developing thymus. However, the role of Ca 2+ signalling in early T-lymphocyte development is not well understood. Here we show that the inositol triphosphate receptors (IP 3 Rs) Ca 2+ ion channels are required for proliferation, survival and developmental progression of T-lymphocyte precursors. Our studies indicate that signalling via IP 3 Rs represses Sox13 , an antagonist of the developmentally important transcription factor Tcf-1 . In the absence of IP 3 R-mediated Ca 2+ signalling, repression of key Notch transcriptional targets—including Hes1 —fail to occur in post β-selection thymocytes, and mice develop aggressive T-cell malignancies that resemble human T-cell acute lymphoblastic leukemia (T-ALL). These data indicate that IP 3 R-mediated Ca 2+ signalling reinforces Tcf-1 activity to both ensure normal development and prevent thymocyte neoplasia. Development of αβ T cells in the thymus proceeds through a highly ordered series of developmental stages, beginning with immature double-negative (DN) thymocytes that lack expression of CD4 and CD8 co-receptors [1] . DN thymocytes represent the most immature thymocyte population and can be further subdivided into four distinct subsets based on CD25 and c-Kit expression: CD25 − c-Kit + (DN1), CD25 + c-Kit + (DN2), CD25 + c-Kit − (DN3) and CD25 − c-Kit − (DN4). DN1 thymocytes represent the earliest T-cell progenitors in the thymus and give rise to DN2 cells. Expansion and proliferation of these early T-cell progenitors is controlled independently of the T-cell receptor (TCR) through cytokine and Notch receptor signalling. As T cells transit from the DN2 to DN3 stage, T-lineage commitment is complete and rearrangement of the TCRβ locus is initiated. At DN3, thymocytes that have generated a functional TCRβ chain capable of pairing with both the CD3 signalling complex and surrogate pre-Tα chain form the pre-TCR complex, and receive specific survival and proliferation signals required for further developmental progression [1] . This requirement, known as the β-selection checkpoint, represents the first checkpoint in T-cell development. Pre-TCR signals drive developmental progression of DN4 thymocytes to CD8 + immature single-positive (ISP) thymocytes, a highly proliferative population that will give rise to CD4 + CD8 + double-positive (DP) thymocytes. On reaching the DP stage, T cells undergo TCRα rearrangement and a series of selection events, culminating in differentiation of DP thymocytes into mature CD4 + or CD8 + single-positive (SP) T cells. Calcium is a universal second messenger in all eukaryotic cells, including T lymphocytes [2] . In resting T cells, concentration of free intracellular Ca 2+ is maintained at low levels. Engagement of TCR results in rapid increase of intracellular Ca 2+ through recruitment and activation of phospholipase Cγ. In T cells, activated phospholipase Cγ1 generates the soluble second messenger inositol-1,4,5-triphosphate,which—on binding the inositol-1,4,5-triphosphate receptor (IP 3 R) on the endoplasmic reticulum (ER) membrane—causes the release of Ca 2+ from the ER into the cytoplasm. Released ER Ca 2+ activates calcium release-activated Ca 2+ (CRAC) channels on the plasma membrane, allowing for sustained influx of extracellular Ca 2+ into the cell. Calcium signals are essential for diverse functions in T cells, including differentiation, TCR-mediated proliferation and cytokine production, and expression of downstream target genes. The importance of sustained Ca 2+ influx in peripheral T cells is emphasized by the severe combined immunodeficiency associated with defects in CRAC channel activity [3] , [4] , [5] . However, conventional αβ T-cell development appears normal in mice where CRAC channel activity is abolished, suggesting that sustained Ca 2+ influx via CRAC channels does not contribute to thymic αβ T-cell development [6] , [7] , [8] , [9] . The role for Ca 2+ signalling at late stages of thymocyte development is well established; several pathways are activated downstream of Ca 2+ , including calcineurin-nuclear factor of activated T-cell, protein kinase C (PKC), nuclear factor- κB (NF-κB) and CaMK-CREB, which are required for DP thymocytes to differentially respond to positive and negative selection signals and for the transition to SP T cells [2] , [10] , [11] , [12] , [13] , [14] . Signalling through the pre-TCR complex results in mobilization of intracellular Ca 2+ stores through Plcγ1, and has been implicated in pre-TCR signalling and early T-cell development [15] , [16] . Consistent with a role for Ca 2+ in pre-TCR signalling, Ca 2+ -dependent signalling pathways such as calcineurin-nuclear factor of activated T-cell, PKCα and NF-κB influence T-cell development and survival from the DN3 stage onwards. Perturbation of individual Ca 2+ -dependent pathways, however, has resulted in relatively modest phenotypic effects. Conditional deletion of calcineurin partially inhibits T-cell development at the DN3 stage, although this phenotype can only be observed in a competitive transplant setting; T-lymphocyte development proceeds normally up to the DP stage in mice with calcineurin-deficient thymocytes [17] , [18] . In fetal thymic organ cultures, defects in pre-TCR + thymocyte survival are observed on PKC inhibition and overexpression of a kinase-dead PKCα enzyme impedes DN to DP transition [19] . However, loss of PKCα or PKCβ alone does not alter thymocyte development, suggesting possible functional redundancy of these proteins [20] . Whether disruption of PKC activity impairs T-cell differentiation or simply reduces thymocyte survival through the decreased production of DP cells has yet to be established. Similarly, inhibition of NF-κB in transgenic mice modestly reduces DN thymocyte numbers, but does not disrupt their differentiation [21] , [22] . Thus, the role of pre-TCR Ca 2+ signalling in thymocyte development remains unclear. Furthermore, physiological mechanisms that influence or control Ca 2+ release downstream of the pre-TCR have yet to be fully elucidated [6] , [8] , [23] , [24] . In this study, we investigated the role of Ca 2+ signalling in early thymocyte development by examining the requirement for IP 3 Rs throughout the DN to DP transition. The IP 3 R is a Ca 2+ permeable ion channel encoded by a family of three genes [25] ( Itpr1 , Itpr2 and Itpr3 ). Functional redundancy between IP 3 Rs and postnatal mortality in the absence of single and multiple Itpr genes has been observed [26] , [27] . IP 3 R channels are functionally diverse; different cells and tissues use distinct IP 3 Rs to regulate specific biological functions [28] . In the thymus, all three IP 3 R subtypes are expressed, suggesting potentially redundant functions between isoforms. To investigate the role of IP 3 Rs in early thymocyte development, we used Tie2-Cre to conditionally ablate all three genes encoding IP 3 Rs. Thymocyte development up to the DP stage was normal in mice with single or double deletion of any of the IP 3 R genes. However, in triple knockout mice, thymocyte development was arrested at DN4 and ISP stages. We identified Sox13, an antagonist of the Wnt transcription factor Tcf-1 that is essential for DN thymocyte differentiation, as a target of pre-TCR Ca 2+ signalling. In the absence of IP 3 R signalling, Sox13 expression is maintained beyond the DN3 stage, thereby disrupting Tcf-1 function and thymocyte development through the DN to DP transition. Furthermore, we identified a role for pre-TCR Ca 2+ signalling in repression of the oncogenic Notch1 transcriptional target Hes1. In concert with this, IP 3 R triple knockout mice rapidly developed thymic tumours that disseminated throughout the body, in a manner reminiscent of T-cell acute lymphoblastic leukemia (T-ALL). The observation that Ca 2+ signals act in early T cells to inhibit transformation demonstrates a new and unexpected role for Ca 2+ signalling in the suppression of leukemogenesis, contrary to its known role in the survival and maintenance of T-ALL [29] . Our findings identify a clear requirement for pre-TCR Ca 2+ signalling through IP 3 R in early lymphocyte development, and provide strong evidence for a dual role of IP3R Ca 2+ signalling in both promoting normal thymocyte development through the DN to DP transition, and in restraining malignant transformation. Role of IP 3 R-Ca 2+ signalling in thymocyte development We examined the requirement for IP 3 R signalling in T-cell development by generating conditional Itpr single-, double- and triple-knockout mice driven by Tie2-Cre, which mediates excision before the DN1 stage of thymocyte development [30] . Itpr2 conditional and null alleles have been described previously [31] , and mice with conditional loxP-flanked alleles for Itpr1 or Itpr3 were generated as described in Supplementary Fig. 1 . Itpr triple-knockout mice were generated as either Itpr1 fl/fl Itpr2 fl/fl Itpr3 fl/fl Tie2 -Cre triple floxed mice (IP 3 R-TKO) or Itpr1 fl/fl Itpr2 −/− Itpr3 fl/fl Tie2 -Cre double floxed and single null mice (DFNKO). Unless stated otherwise, control mice used throughout the remainder of the manuscript were Itpr1 fl/fl Itpr2 fl/fl Itpr3 fl/fl . IP 3 R-TKO and IP 3 R-DFNKO mice were born at expected Mendelian ratios. As no phenotypic differences were observed between IP 3 R-TKO and IP 3 R-DFNKO, we used IP 3 R-TKO mutant mice for further investigation ( Fig. 1a and Supplementary Fig. 3 ). IP 3 R-TKO mice, but not single- or double-knockout mice, displayed severe defects in early thymocyte development ( Fig. 1 and Supplementary Fig. 2a ). Severe reduction of Itpr in IP 3 R-TKO thymocytes was confirmed by western blot analysis ( Supplementary Fig. 2b ). Ca 2+ influx in response to TCR cross-linking with an anti-CD3 antibody was also significantly impaired ( Supplementary Fig. 2c ). 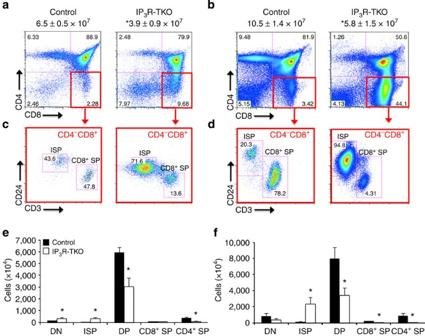Figure 1:IP3R-Ca2+store depletion promotes the DN to DP transition. Expression of surface CD4 and CD8 (top row) in 1-week-old neonate (a) and 6-week-old adult (b) thymi of IP3R-TKO and control mice. Total thymic cellularity is shown above plots (mean±s.e.m.). CD8+CD4−thymocytes were subgated (red boxes) and examined for surface expression of CD24 and CD3 to observe ISP cells contained in the CD8+CD4−populations shown inaandb. This was done in both neonatal (c) and adult (d) thymi of IP3R-TKO and control mice. Numbers in plots indicate percentage of cells. Absolute cellularity as depicted ina–dfor neonatal (e) and (f) adult thymic subsets (mean±s.e.m.). All animals displaying signs of malignant disease were excluded from these analyses. Data are representative of a minimum of five (a–f) independent experiments. *P<0.05, measured with two-tailed Student’st-test. Figure 1: IP 3 R-Ca 2+ store depletion promotes the DN to DP transition. Expression of surface CD4 and CD8 (top row) in 1-week-old neonate ( a ) and 6-week-old adult ( b ) thymi of IP 3 R-TKO and control mice. Total thymic cellularity is shown above plots (mean±s.e.m.). CD8 + CD4 − thymocytes were subgated (red boxes) and examined for surface expression of CD24 and CD3 to observe ISP cells contained in the CD8 + CD4 − populations shown in a and b . This was done in both neonatal ( c ) and adult ( d ) thymi of IP 3 R-TKO and control mice. Numbers in plots indicate percentage of cells. Absolute cellularity as depicted in a – d for neonatal ( e ) and ( f ) adult thymic subsets (mean±s.e.m.). All animals displaying signs of malignant disease were excluded from these analyses. Data are representative of a minimum of five ( a – f ) independent experiments. * P <0.05, measured with two-tailed Student’s t -test. Full size image IP 3 R-TKO thymi were noticeably smaller, with a consistent reduction in cellularity as compared with those of littermate controls ( Fig. 1a,b ). The distribution of thymocyte subsets was also abnormal. In IP 3 R-TKO neonates, there was a significant increase in both DN and CD8 + CD3 − CD24 + ISP T cells, a transient progenitor cell present between the DN to DP transition ( Fig. 1a,c ). Numbers of DP thymocytes were reduced by 50% and a significant reduction in mature CD4 + SP thymocytes was also observed. Mature CD8 + SP thymocytes were present in numbers similar to controls. Developing T lymphocytes can be divided into two major lineages: αβ or γδ, which refer to the different TCR genes that have undergone somatic recombination. To address whether the increase in DN thymocytes in IP 3 R-TKO mice resulted from aberrations in a specific lineage, we analysed expression of CD3, CD24 and γδ TCR in DN thymocytes ( Supplementary Fig. 4a,b ). γδ T-cell numbers were reduced fourfold in IP 3 R-TKO thymi ( Supplementary Fig. 4c ), indicating that development of γδ T-cell lineage subsets was also impaired in IP 3 R-TKO mice. Examination of thymocyte development in young adult IP 3 R-TKO mice (6 weeks) revealed further accumulation of ISP T cells and compensatory reduction in DP thymocytes ( Fig. 1b,d ). Together, these data demonstrated a requirement for IP 3 R-mediated Ca 2+ signalling during development of both αβ and γδ T-cell lineages, highlighting a critical role for pre-TCR-mediated Ca 2+ store depletion in thymocytes throughout the DN to DP transition. IP 3 R-Ca 2+ loss impairs thymocyte proliferation and survival To further characterize the developmental defect observed at the DN stage in IP 3 R-TKO neonates, we examined the lineage-negative thymocyte distribution between DN1 to DN4 stages. Successful rearrangement and expression of intracellular TCRβ can be detected between DN2 and DN3. This process, also known as the β-selection checkpoint, is required for T-cell development to progress beyond the DN3 stage [32] . Although numbers of DN3 thymocytes were only slightly elevated when compared with controls, IP 3 R-TKO mice displayed a marked increase in DN4 thymocytes ( Fig. 2a,b ). We next examined expression of TCRβ in pre- and post-β-selection thymocytes. Expression of intracellular TCRβ in IP 3 R-TKO DN3 and DN4 thymocytes was similar to controls ( Fig. 2c ). Together, these data indicated that IP 3 R-Ca 2+ was not required for TCRβ rearrangement or expression. 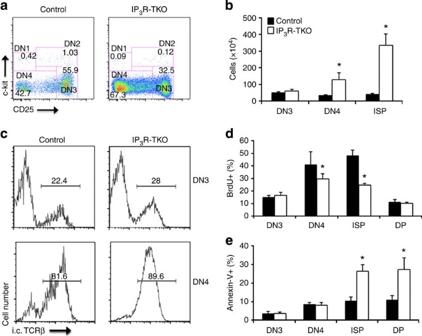Figure 2:IP3R-Ca2+store depletion promotes pre-TCR-mediated proliferation and survival. (a) Lineage−thymocytes of 1-week-old neonate control and IP3R-TKO mice were examined for surface c-Kit and CD25 surface expression to determine DN3 and DN4 T-cell subsets. (b) Total cellularity of populations depicted ina(mean±s.e.m.). ISP thymocyte cellularity was determined as inFig. 1. (c) Intracellular TCR-β (i.c. TCRβ) chain expression in DN3 (top panels) and DN4 (bottom panels) thymocytes of neonatal control and IP3R-TKO mice. Cell number is expressed as percentage of total population depicted. (d) Thymocyte proliferation as measured by BrdU incorporation. (e) Apoptosis as measured by Annexin-V staining for neonatal control and IP3R-TKO mice. All animals displaying signs of malignant disease were excluded. Data are representative of a minimum of three independent experiments. *P<0.05, measured with two-tailed Student’st-test. Figure 2: IP 3 R-Ca 2+ store depletion promotes pre-TCR-mediated proliferation and survival. ( a ) Lineage − thymocytes of 1-week-old neonate control and IP 3 R-TKO mice were examined for surface c-Kit and CD25 surface expression to determine DN3 and DN4 T-cell subsets. ( b ) Total cellularity of populations depicted in a (mean±s.e.m.). ISP thymocyte cellularity was determined as in Fig. 1 . ( c ) Intracellular TCR-β (i.c. TCRβ) chain expression in DN3 (top panels) and DN4 (bottom panels) thymocytes of neonatal control and IP 3 R-TKO mice. Cell number is expressed as percentage of total population depicted. ( d ) Thymocyte proliferation as measured by BrdU incorporation. ( e ) Apoptosis as measured by Annexin-V staining for neonatal control and IP 3 R-TKO mice. All animals displaying signs of malignant disease were excluded. Data are representative of a minimum of three independent experiments. * P <0.05, measured with two-tailed Student’s t -test. Full size image Rag2 −/− T cells lack the recombination machinery necessary for TCRβ recombination and thus cannot generate a functional pre-TCR. As a result, Rag2 −/− T cells are arrested at DN3. This arrest represents an important developmental checkpoint in T-cell development known as β-selection, and acts to prevent uncontrolled proliferation and malignancy in the thymus. As we observed a significant accumulation of thymocytes in IP 3 R-TKO mice, we next askedwhether, in the absence of Itpr , thymocytes were able to bypass the β-selection checkpoint. To do this, we crossed IP 3 R-TKO mice onto a Rag2 −/− genetic background [33] and examined thymocyte development. T-cell development was completely blocked at the DN3 stage in Rag2 −/− IP 3 R-TKO thymi, indicating that the β-selection checkpoint remained intact in the absence of pre-TCR-mediated Ca 2+ store depletion ( Supplementary Fig. 5 ). We next set out to elucidate the cause of decreased thymic cellularity and accumulation of DN4 and ISP thymocytes in neonatal IP 3 R-TKO mice. Decreased thymic cellularity can be the result of reduced proliferation or increased cell death. IP 3 R-TKO thymocyte proliferation was modestly reduced at both DN4 and ISP stages ( Fig. 2d ). In agreement with previous studies linking pre-TCR Ca 2+ signalling and thymocyte survival [17] , [21] , we observed a significant increase in apoptosis at the ISP stage in IP 3 R-TKO mice ( Fig. 2e ). DP thymocyte apoptosis was also significantly increased ( Fig. 2e ). Taken together, these data strongly suggested that the decrease in thymic cellularity observed in neonatal IP 3 R-TKO mice was a combined result of both impaired thymocyte survival and proliferation, and that accumulation of DN4 and ISP thymocytes was not a result of a survival advantage or uncontrolled proliferation. These data also demonstrated that IP 3 R-Ca 2+ was required for thymocyte survival at the ISP to DP transition and was essential for proliferation in pre-TCR + DN4 and ISP thymocytes. Observed increased numbers of thymocytes at the DN4 and ISP stages was initially puzzling, as we also observed decreased survival and proliferation. We postulated that developmental arrest of thymocytes transitioning to DN4 and ISP stages might result in excessive thymocyte accumulation/trapping at these stages, which might be only partially counteracted by observed increases in apoptosis and reductions in proliferation, still resulting in overall increased numbers of thymocytes. In support of this, examination of T-cell development in E17.5 thymi, where a synchronous wave of precursors can be observed [34] , demonstrated that IP 3 R-TKO thymocytes significantly accumulated at DN4 and ISP stages, consistent with a block to thymocyte progression through post-selection stages ( Supplementary Fig. 6a,d,e ). Thus, accumulation of cells at DN4 and subsequent ISP stages occurs as thymocytes are significantly blocked in their transition to the DP stage. Observed increased apoptosis and reduced proliferation are not sufficient to overcome this accumulation, resulting in an overall increase in thymocyte cell numbers at these stages. Tie2-Cre is active in both haematopoietic and endothelial lineages present in the thymus. To address the thymocyte-autonomous nature of the developmental block observed in vivo , we performed experiments on cultured T cells by sorting Sca-1 + fetal liver haematopoietic stem and progenitor cells on OP9 stromal cells expressing the Notch ligand Delta-1 (OP9-DL1), which allows in vitro differentiation of T cells up to the DP stage. In contrast to littermate controls, IP 3 R-TKO cells were impaired in progression to the DP stage, accumulating at DN and recapitulating the block to differentiation observed in vivo ( Supplementary Fig. 6b,c ). To further investigate the thymocyte autonomous requirement for IP 3 Rs, we used CD4-Cre, active at the beginning of the DN3 stage [35] , to ablate all three isoforms of IP 3 R. The phenotype of this knockout closely resembled that of mice with Tie2-Cre ablation of all three isoforms of IP 3 R, causing early mortality due to thymic tumours ( Supplementary Fig. 7 ). Collectively, these data identified a cell-autonomous requirement for IP 3 R-Ca 2+ at the β-selection checkpoint and in pre-TCR-mediated differentiation, survival and proliferation of αβ T cells. IP 3 R-Ca 2+ reinforces αβ T-cell lineage gene regulation Although our data demonstrated that pre-TCR Ca 2+ was essential for the DN4 to DP transition, genes and pathways regulated by Ca 2+ at these stages have not been identified. To address this, we performed an exploratory global gene expression analysis in ISP thymocytes isolated from IP 3 R-TKO and control thymi ( Fig. 3a ). We identified 955 differentially expressed genes at the ISP stage. KEGG (Kyoto Encyclopedia of Genes and Genomes) pathway analysis of differentially expressed genes revealed involvement in focal adhesion, extracellular matrix–receptor interactions, tight junctions, endocytosis and phosphatidylinositol-, mitogen-activated protein kinase (MAPK)- and calcium-signalling pathways ( Fig. 3b and Supplementary Tables 1 and 2 ). Changes in ER Ca 2+ and other adverse conditions can impair the formation of new proteins, resulting in ER stress [36] . To investigate the potential impact of ER stress on observed phenotypes, we examined our microarray data for any upregulation of ER stress-responsive genes, including ATF2 , ATF4 , SERCA and CHOP . None of these genes were differentially expressed in IP 3 R-TKO thymocytes (microarray data deposited on the NIH Gene Expression Omnibus at http://www.ncbi.nlm.nih.gov/geo/ (GSE57997)). 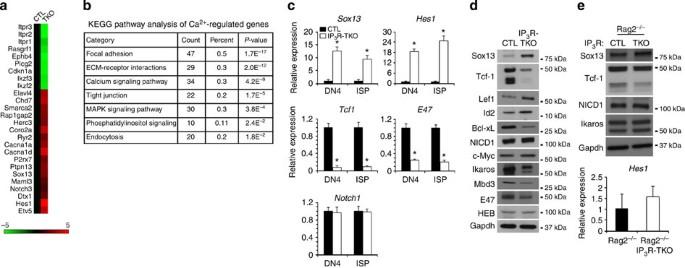Figure 3: Deregulation of gene expression in the absence of IP3R-Ca2+. (a) Heat map for a subset of genes in neonatal IP3R-TKO and control (CTL) ISP T cells. Three biological replicates of IP3R-TKO and control ISP T cells were pooled and used for analysis. Control ISP cells were used as baseline; green denotes genes downregulated in TKO compared with control and red denotes upregulation of these genes. (b) KEGG analysis for functional pathways regulated by IP3R-Ca2+with a threefold threshold of differential expression (seeSupplementary Tables 1 and 2for additional pathway analyses). (c) qRT–PCR forSox13,Hes1,Notch1,Tcf-1andE47expression in neonatal control (black bars) and IP3R-TKO (white bars) sorted ISP thymocytes. Data represent three biological replicates. Bars represent s.d. and error bars were measured by the non-parametric Wilcoxon signed rank sum (two-group) test. Sorting gates are based onFig. 1. (d) Western blot analysis of ED 17.5 total thymocyte lysates from control (CTL) and IP3R-TKO mice. Cleaved intracellular Notch1 (NICD1). (e) Western blot analysis (top) and qRT–PCR forHes1expression (bottom) of 6-week-old control and IP3R-TKO total thymocytes on a Rag2−/−background. All animals displaying signs of malignant disease were excluded from these analyses. *P<0.05, measured with two-tailed Student’st-test. Figure 3: Deregulation of gene expression in the absence of IP 3 R-Ca 2+ . ( a ) Heat map for a subset of genes in neonatal IP 3 R-TKO and control (CTL) ISP T cells. Three biological replicates of IP 3 R-TKO and control ISP T cells were pooled and used for analysis. Control ISP cells were used as baseline; green denotes genes downregulated in TKO compared with control and red denotes upregulation of these genes. ( b ) KEGG analysis for functional pathways regulated by IP 3 R-Ca 2+ with a threefold threshold of differential expression (see Supplementary Tables 1 and 2 for additional pathway analyses). ( c ) qRT–PCR for Sox13 , Hes1 , Notch1 , Tcf-1 and E47 expression in neonatal control (black bars) and IP 3 R-TKO (white bars) sorted ISP thymocytes. Data represent three biological replicates. Bars represent s.d. and error bars were measured by the non-parametric Wilcoxon signed rank sum (two-group) test. Sorting gates are based on Fig. 1 . ( d ) Western blot analysis of ED 17.5 total thymocyte lysates from control (CTL) and IP 3 R-TKO mice. Cleaved intracellular Notch1 (NICD1). ( e ) Western blot analysis (top) and qRT–PCR for Hes1 expression (bottom) of 6-week-old control and IP 3 R-TKO total thymocytes on a Rag2 −/− background. All animals displaying signs of malignant disease were excluded from these analyses. * P <0.05, measured with two-tailed Student’s t -test. Full size image The expression of several genes critical to T-cell development was significantly altered, including increased expression of Sox13 and the Notch transcriptional target Hes1 . Alterations in messenger RNA expression of these genes in IP 3 R mutants was confirmed by quantitative reverse transcription–PCR (qRT–PCR) analyses of RNA extracted from purified neonatal ISP cells from controls and mutants ( Fig. 3c ). Sox13 is a γδ-T-cell lineage-restricted transcription factor that opposes development of αβ T cells by antagonizing the high mobility group box transcription factor Tcf-1 (Tcf7) [37] . Tcf-1 is essential for differentiation and survival of thymocytes through the DN to DP transition, and its expression is rapidly increased on pre-TCR signalling [38] . As phenotypes of Sox13 Tg and Tcf-1 −/− mice resemble that of our IP 3 R-TKOs, we examined expression of Sox13 and Tcf-1 by western blot analysis. In agreement with gene expression data, Sox13 was significantly increased in ED 17.5 IP 3 R-TKO thymocytes, the majority of which are transitioning to the DP stage, and Tcf-1 expression was nearly absent ( Fig. 3c,d ). Importantly, expression of Tcf-1 and Sox13 proteins was similar in Rag2 −/− IP 3 R-TKO and Rag2 −/− thymocytes, which lack a functional pre-TCR and are arrested at the β-selection checkpoint, demonstrating that IP 3 R-Ca 2+ influences expression of these proteins following β-selection ( Fig. 3e ). In thymocytes, Tcf-1 functions as both a transcriptional activator and repressor through interactions with β-catenin. At the DN stage, Tcf-1 acts to repress Lef1 and Id2 (refs 39 , 40 ), and is essential for mediating DP thymocyte survival by increasing expression of the pro-survival protein Bcl-x L [41] . Similar to Tcf-1 −/− mice, we observed elevated expression of Lef1 and Id2 in IP 3 R-TKO thymocytes and decreased amounts of Bcl-x L , consistent with diminished Tcf-1 function. Together with our IP 3 R loss-of-function studies, these data indicated a requirement for IP 3 R-mediated Ca 2+ release downstream of pre-TCR in establishing a gene regulatory programme in post β-selected thymocytes, whereby Ca 2+ signalling acts to reinforce differentiation and survival of αβ T-cell lineage by repressing Sox13, thus enabling upregulation of Tcf-1 post β-selection. Notch signalling is required for T-lineage specification and commitment [42] , [43] , [44] . Moreover, Notch and pre-TCR signals collaborate in mediating differentiation, proliferation and survival of T cells through the β-selection checkpoint [45] , [46] . Of note, Notch signalling is repressed in T cells following β-selection, which is mediated through Tcf-1 and the Ikaros-NuRD chromatin-remodelling complex [47] , [48] , [49] . Our microarray analysis of IP 3 R-TKO ISP cells revealed upregulation of a subset of Notch target genes in mutant ISP cells compared with controls, including Hes1 , suggesting potential dysregulation of Notch signalling pathways. Our microarray analyses had indicated no changes in Notch1 gene expression in neonatal ISP cells of mutants relative to controls, a result confirmed by qRT–PCR analyses ( Fig. 3c ). To further investigate potential increased activation of Notch1 in IP 3 R-TKO thymi, expression of cleaved intracellular Notch1 (NICD1) was examined by western blot analyses of fetal thymi, and was found to be unchanged between IP 3 R-TKO and controls ( Fig. 3d ). Together, these observations suggest that a subset of Notch1 target genes were upregulated in the absence of activated Notch1. Alternatively, expression of genes involved in repression of the Notch signalling pathway might be altered. Tcf-1 negatively regulates expression of Notch1 and its target genes in T-lineage-committed thymocytes. In IP 3 R-TKO thymocytes, Tcf-1 expression and activity were significantly impaired ( Fig. 3c,d ). Thus, activation of Notch1 target genes, such as Hes1 , may be accounted for by decreased expression of Tcf-1 observed in IP 3 R-TKO thymocytes. Expressions of genes associated with the Ikaros-NuRD complex, a transcriptional repressor of Notch signalling, were also altered. Ikaros (Ikzf1) protein levels were severely reduced in ED 17.5 IP 3 R-TKO thymocytes ( Fig. 3d ). Mbd3, a central component of the NuRD chromatin-remodelling complex required for NuRD-Hdac interaction [50] , was reduced in mutants relative to controls ( Fig. 3d ). The E protein E47 (Tcf3) positively regulates expression of Notch1 and is antagonized by Id proteins at the β-selection checkpoint [51] . However, E47 mRNA and protein expression were reduced in IP 3 R-TKO thymocytes ( Fig. 3c,d ). The E protein HEB is also required for the DN to DP transition, and its loss-of-function leads to a developmental block at the ISP stage [52] . In contrast to E47, HEB protein levels in IP 3 R-TKO were similar to those of controls ( Fig. 3d ). Consistent with IP 3 R-Ca 2+ influencing Notch target gene expression after TCRβ recombination, expression of Tcf-1, Ikaros, cleaved NICD1 protein and Hes1 mRNA in Rag2 −/− IP 3 R-TKO was similar to Rag2 −/− thymocytes ( Fig. 3d ). Taken together, these results indicated a requirement for IP 3 R-mediated Ca 2+ signalling in post β-selected thymocytes to repress Notch target gene expression, probably through positive regulation of the Ikaros-NuRD complex gene expression and repression of the Tcf-1 antagonist Sox13. Impaired survival and development of T-ALL in IP 3 R-TKO mice IP 3 R-TKO and IP 3 R-DFNKO mice developed thymic hyperplasia beyond 6 weeks of age ( Fig. 4a ), followed by the appearance of massive thymic tumours. Thymic tumours in TKO mice were fully penetrant by 12 weeks of age, and resembled localized T-cell lymphoblastic lymphoma (T-LBL) [53] ; tumour invasion into adjacent tissues was observed in the absence of disseminated disease ( Fig. 4a ). Beyond 12 weeks, we observed significant morbidity and mortality ( n >100, IP 3 R-TKO; Fig. 4b ), concomitant with significant lymphoblast infiltration of peripheral blood, bone marrow and spleen ( Fig. 4c and Supplementary Fig. 8 ). At this stage, tumours were transplantable, indicating that loss of Itpr intrinsically in thymocytes leads to the development of malignant disease. 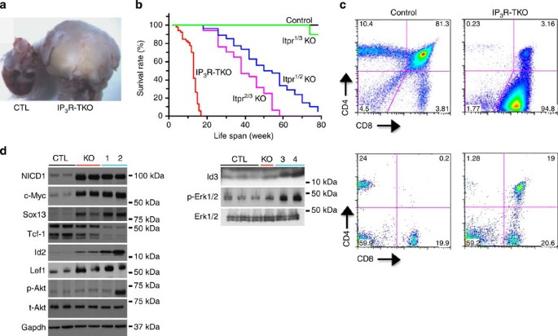Figure 4:Development of T-ALL in the absence of Itpr-Ca2+. (a) Thymus of adult tumour-bearing IP3R-TKO mouse (right) compared with control thymus (CTL, left). (b) Kaplan–Meier survival curve of double and triple Itpr knockout lines (n>100, IP3R-TKO).Itpr1fl/−Itpr3−/−Tie2-Cre (Itpr1/3KO),Itpr1fl/flItpr2−/−Tie2-Cre (Itpr1/2KO) orItpr2fl/−Itpr3fl/flTie2-Cre (Itpr2/3KO). (c) Surface CD4 and CD8 expression of control and T-ALL burdened thymi (top) and peripheral blood (bottom) of IP3R-TKO adult animals. (d) Western blotting of cleaved intracellular Notch1 (NICD1), c-Myc, Tcf-1, Sox13, Lef1, Id2, Id3, and total and phosphorylated Erk and Akt in adult control and IP3R-TKO hyperplastic (KO), T-LBL (1, 3) and T-ALL (2, 4) burdened thymi. Data are representative of a minimum of ten (a,c), three (d) and one (b) independent experiments. Hyperplasia, T-LBL and T-ALL were defined by the presence of disease and the extent of extra-thymic tissue involvement. Age was not used to define these stages, as we observed significant variability in the age of onset and age of progression from hyperplasia to T-LBL to T-ALL in IP3R-TKO mice. Figure 4: Development of T-ALL in the absence of Itpr-Ca 2+ . ( a ) Thymus of adult tumour-bearing IP 3 R-TKO mouse (right) compared with control thymus (CTL, left). ( b ) Kaplan–Meier survival curve of double and triple Itpr knockout lines ( n >100, IP 3 R-TKO). Itpr1 fl/− Itpr3 −/− Tie2 -Cre (Itpr 1/3 KO), Itpr1 fl/fl Itpr2 −/− Tie2 -Cre (Itpr 1/2 KO) or Itpr2 fl/− Itpr3 fl/fl Tie2 -Cre (Itpr 2/3 KO). ( c ) Surface CD4 and CD8 expression of control and T-ALL burdened thymi (top) and peripheral blood (bottom) of IP 3 R-TKO adult animals. ( d ) Western blotting of cleaved intracellular Notch1 (NICD1), c-Myc, Tcf-1, Sox13, Lef1, Id2, Id3, and total and phosphorylated Erk and Akt in adult control and IP 3 R-TKO hyperplastic (KO), T-LBL (1, 3) and T-ALL (2, 4) burdened thymi. Data are representative of a minimum of ten ( a , c ), three ( d ) and one ( b ) independent experiments. Hyperplasia, T-LBL and T-ALL were defined by the presence of disease and the extent of extra-thymic tissue involvement. Age was not used to define these stages, as we observed significant variability in the age of onset and age of progression from hyperplasia to T-LBL to T-ALL in IP 3 R-TKO mice. Full size image Progression of advanced T-LBL to T-ALL is marked by a transition of bone marrow to include ≥25% immature lymphoblasts, which was frequently observed in moribund IP 3 R-TKO. Post-mortem histological examination also revealed leukocyte infiltration into non-lymphoid organs, including the lungs and liver ( Supplementary Fig. 9 ). Lymphoid blasts in the thymus and peripheral blood were CD8 + CD3 − CD24 hi and expressed intracellular TCR-β with variable expression of CD4, consistent with cells being arrested at ISP and DP stages ( Fig. 4c ). We also observed a progressive decrease in survival beginning at 6 months of age in Itpr1 fl/fl Itpr2 −/− Tie2 -Cre and Itpr2 fl/− Itpr3 fl/fl Tie2 -Cre mice, but thymic tumours were not observed on post-mortem examination. Itpr1 fl/fl Itpr2 −/− Tie2 -Cre and Itpr2 fl/ − Itpr3 fl/fl Tie2- Cre mice showed no evidence of haematologic malignancy when examined before 6 months of age by flow cytometry of peripheral blood. In addition, deceased Itpr1 fl/fl Itpr2 −/− Tie2 -Cre and Itpr2 fl/ − Itpr3 fl/fl Tie2- Cre mice showed no evidence of haematologic malignancy in the spleen or the gastrointestinal tract. The cause of lethality in these mice remains to be determined. Together, these findings suggested that the loss of all three Itpr genes leads to development of an aggressive T-LBL corresponding to the ISP stage of development that rapidly disseminates and progresses to T-ALL. Activating mutations in Notch1 have been implicated in development of both T-LBL and T-ALL in mice and humans [54] . As post β-selected thymocytes in IP 3 R-TKO mice failed to repress key Notch signalling targets, we examined Notch1 activity in tumour-burdened adult thymi. In contrast to fetal IP 3 R-TKO thymocytes, NICD1 was significantly increased in adult IP 3 R-TKO hyperplastic and tumour-burdened thymi when compared with littermate controls ( Fig. 4d ). In addition, sequencing of Notch1 complementary DNA revealed mutations in the proline, glutamic acid, serine, threonine-rich (PEST) domain (coded by exon 34), which are commonly associated with human T-ALLs and murine T-cell lymphomas ( Table 1 and Supplementary Fig. 10 ) [39] , [55] , [56] , [57] . In total, ten cDNA clones were obtained from three individual leukemic animals. Out of 30 clones sequenced, 14 had mutations in exon 34. These observed mutations are predicted to alter the protein sequence of Notch1 to result in truncated proteins and loss of the PEST domain ( Table 1 and Supplementary Fig. 10 ). In vitro studies indicate that truncation or deletion of the PEST domain of Notch1 result in a prolonged half-life of NICD1 and increased Notch1 signalling [58] . Together, these data suggested that in contrast to pre-leukemic IP 3 R-TKO thymocytes that had normal levels of NICD1, leukemic T cells had increased Notch1 signalling caused by activating mutations of Notch1. Table 1 Mutations identified in exon 34 of the mouse Notch1 gene in IP3R-TKO thyme. Full size table The proto-oncogene c-Myc is an important transcriptional target of Notch1 that contributes to development and growth of both T-LBL and T-ALL [53] . In IP 3 R-TKO fetal thymocytes, c-Myc expression was similar to that of controls. However, in mutant adult thymi, c-Myc overexpression was coincident with hyperplasia ( Fig. 4d ), consistent with c-Myc activation being a critical early event in Notch1-mediated oncogenesis [59] . Oncogenic activation of Notch signalling in T-ALL is also associated with increased Ras-Mapk and PI3K-Akt activity [60] . Therefore, we examined the phosphorylation status of Erk and Akt. Erk phosphorylation was increased in the majority of tumours examined, but not at the onset of thymic hyperplasia in adult IP 3 R-TKO ( Fig. 4d ). In contrast, Akt phosphorylation was increased only in animals where disease had spread outside the thymus and into adjacent tissues and bone marrow, in agreement with previous studies linking PI3K-Akt activation and the progression of T-LBL to T-ALL [53] . Deletions in TCF-1 have been reported in a subset of paediatric T-ALLs that resemble early thymic progenitors (ETP-ALL) and this subtype is associated with diminished expression of TCF-1 (refs 39 , 40 ). Tcf-1 −/− mice succumb to precursor T-cell lymphomas that resemble human T-ALL, consistent with Tcf-1 being a classical tumour suppressor. The development of T-cell lymphomas in Tcf-1 −/− mice is dependent on high Lef1 expression, as Lef1 deletion significantly delayed or prevented malignant transformation. Based on the observation that IP 3 R-TKO fetal thymocytes displayed aberrant upregulation of the Tcf-1 antagonist Sox13, and lack significant Tcf-1 expression, we investigated if Tcf-1 function was impaired in adult IP 3 R-TKO tumours. Tcf-1 protein was severely diminished in tumour-burdened but not hyperplastic adult IP 3 R-TKO thymi. In contrast, Sox13 was significantly upregulated in adult IP 3 R-TKO thymocytes and displayed a progressive increase in expression as thymi transitioned from marked hyperplasia to overt malignancy ( Fig. 4d ). Consistent with diminished Tcf-1 function in IP 3 R-TKO tumours, Lef1 was uniformly upregulated in hyperplastic and tumour-burdened IP 3 R-TKO thymi. Interestingly, Id2 displayed a stepwise increase in expression as thymi developed marked hyperplasia and transitioned from T-LBL to T-ALL, mirroring the loss of Tcf-1 protein. Increased Id3 expression was also observed in both T-LBL and T-ALL thymic tumours but not in younger adult thymi with only moderate hyperplasia. As Id3 expression appeared normal in IP 3 R-TKO fetal thymocytes, gain of Id3 expression is probably independent of Tcf-1or Sox13. In DN thymocytes, pre-TCR signalling induces rapid cell cycle entry, survival and developmental progression of β-selected thymocytes to the DP stage. Ca 2+ signalling mediated through pre-TCR-induced activation of Plcγ1 is thought to be important for this developmental transition. However, the role of IP 3 R Ca 2+ release in developmental progression of thymocytes in addition to the influence of Ca 2+ signalling on the network of transcription factors that drive T cells through the DN to DP transition has not been addressed. Before this work, understanding of the role of IP 3 R at early stages of T-cell development was limited to studies examining thymocyte progenitor survival in vitro and a single gene knockout study of IP 3 R1 where no defects in thymic development were observed [21] , [61] . Data presented here establish a clear requirement for IP 3 R and Ca 2+ signalling in pre-TCR thymocyte development, and reveal an unexpected role for pre-TCR Ca 2+ signalling in the prevention of lymphoid malignancy. Developmental arrest of thymocytes at DN and ISP stages, accompanied by decreased proliferation and increased apoptosis, was observed in Tie2-Cre knockouts of all three IP 3 Rs. Although we primarily used Tie2-Cre in this manuscript, it is important to note that knockout of all three isoforms of IP 3 R with CD4-Cre, which is active at the beginning of the DN3 stage of thymocyte development [35] , was also performed. This knockout closely phenocopied our results with Tie2-Cre, causing early mortality due to thymic tumours ( Supplementary Fig. 7 ). Further evidence that the observed thymocyte phenotype was cell intrinsic was obtained by our in vitro OP9-DL1 experiments. The developmental phenotype we observed in vivo was faithfully recapitulated in vitro and included disruption of the DN to DP transition, the accumulation of DN and ISP T cells, and loss of DP thymocytes. Together, these observations strongly suggested that the phenotype of the IP 3 R-TKO mice was cell intrinsic to T cells. These phenotypes were not observed in any single or double tissue-specific knockout of IP 3 Rs, suggesting redundancy between the three IP 3 R isoforms. This level of redundancy probably occurs in other cell types in addition to T cells, as most eukaryotic cells express more than one IP 3 R isoform [62] . Functional redundancy of IP 3 Rs in T-cell development is consistent with critical roles of IP 3 R and Ca 2+ throughout the lifespan of T cells. In contrast with the critical role of IP 3 R in early T-cell development, store-operated Ca 2+ entry (SOCE) mediated by STIM1 and STIM2 are dispensable for the development of conventional αβ T cells [9] . It has been proposed that a differential requirement for Ca 2+ signalling exists throughout thymocyte development, where strong and sustained increases in Ca 2+ via SOCE are required late in T-cell maturation, while small localized and transient Ca 2+ release as mediated by the IP 3 R is sufficient, in concert with other ion channels, to promote early thymocyte development and selection. Our data are consistent with this hypothesis and highlight the central role of Ca 2+ throughout thymocyte development. Mutants that exhibit decreased Tcf-1 activity share many aspects of the phenotype exhibited by IP 3 R-TKO thymocytes. Both Tcf-1 mRNA and protein were significantly decreased in fetal and neonatal IP 3 R-TKO thymocytes. In addition, an antagonist of Tcf-1 activity, Sox13, was aberrantly upregulated in IP 3 R-TKO thymocytes after β-selection. Consistent with diminished Tcf-1 activity, IP 3 R-TKO thymocytes displayed significant changes in the expression of key Tcf-1 transcriptional targets, including increased expression of the oncogenic transcription factor Lef-1 and decreased expression of the pro-survival Bcl-2 family member Bcl-x L [39] , [41] . In both IP 3 R-TKO and Tcf-1 mutants, T-cell development is blocked at DN and ISP stages. Thymocyte proliferation is also reduced beginning at the DN stage and thymocyte survival is impaired at both pre-TCR and TCR-dependent stages of T-cell development. Similarly, transgenic mice overexpressing Sox13, an antagonist of Tcf-1, exhibit impaired αβ T-lineage development and DN thymocyte proliferation [37] . The balance of E and Id proteins was also altered in IP 3 R-TKO thymocytes and may also contribute to aspects of the observed phenotypes. The severe block at the ISP stage in IP 3 R-TKO mice resembles defects seen in HEB −/− animals [52] , [63] . Although HEB expression in IP 3 R-TKO T cells was not altered, reduced levels of E47 and increased levels of Id proteins suggest that HEB function is likely to be compromised in IP 3 R-TKO mice. The initial developmental block observed in triple knockout thymocytes is followed by progressive development of an aggressive leukemia resembling T-ALL, demonstrating a previously unappreciated role for IP 3 R signalling in suppressing the development of T-cell leukemia ( Fig. 5b ). Development of T-ALL was observed in all IP 3 R-TKO mice and was detected as early as 6 weeks of age. Similar to the developmental arrest of T lymphocytes, this leukemic phenotype was only observed when all three Itpr genes were ablated. 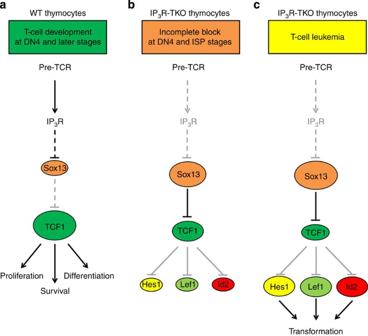Figure 5:A working model for the role of IP3R signalling in early thymocyte development and T-cell malignancy. A working model for the role of IP3R signalling in early thymocyte development and T-cell malignancy based on data presented in this work and that of others37,38,49,54. (a) In wild-type (WT) thymocytes, signalling through the Pre-TCR initiates the release of Ca2+from intracellular stores via IP3Rs. At DN4, IP3R-dependent pathways normally repress transcription of Sox13. In the absence of Sox13, Tcf-1 is active, promoting proliferation, survival and differentiation of T cells37. (b) In the absence of all three isoforms of IP3R, Sox13 expression is significantly elevated and expression of Tcf-1 is significantly reduced. Previous studies have demonstrated that transgenic overexpression of Sox13 and consequent low activity of Tcf-1 results in a block at the DN4 stage, as observed in IP3R TKO thymocytes37,38. Consequent to repression of Tcf-1, targets of Tcf-1 repression, including Hes1, Lef1 and Id2, are upregulated49, as also observed in IP3R TKO thymocytes. (c) At approximately 3 months of age, IP3R-deficient mice develop an aggressive T-cell malignancy resembling human T-cell acute lymphoblastic leukemia (T-ALL) involving multiple genetic events, which includes further upregulation of Sox13, and more severe repression of Tcf-1 (refs37,38). Tumours were also found to express activated forms of Notch1 (ref.54). Therefore, our observation of increased Sox13 and decreased Tcf-1 in IP3R KO thymocytes can account for the abnormal thymocyte development observed in our mutants. Figure 5: A working model for the role of IP 3 R signalling in early thymocyte development and T-cell malignancy. A working model for the role of IP 3 R signalling in early thymocyte development and T-cell malignancy based on data presented in this work and that of others [37] , [38] , [49] , [54] . ( a ) In wild-type (WT) thymocytes, signalling through the Pre-TCR initiates the release of Ca 2+ from intracellular stores via IP 3 Rs. At DN4, IP 3 R-dependent pathways normally repress transcription of Sox13. In the absence of Sox13, Tcf-1 is active, promoting proliferation, survival and differentiation of T cells [37] . ( b ) In the absence of all three isoforms of IP 3 R, Sox13 expression is significantly elevated and expression of Tcf-1 is significantly reduced. Previous studies have demonstrated that transgenic overexpression of Sox13 and consequent low activity of Tcf-1 results in a block at the DN4 stage, as observed in IP3R TKO thymocytes [37] , [38] . Consequent to repression of Tcf-1, targets of Tcf-1 repression, including Hes1, Lef1 and Id2, are upregulated [49] , as also observed in IP 3 R TKO thymocytes. ( c ) At approximately 3 months of age, IP 3 R-deficient mice develop an aggressive T-cell malignancy resembling human T-cell acute lymphoblastic leukemia (T-ALL) involving multiple genetic events, which includes further upregulation of Sox13, and more severe repression of Tcf-1 (refs 37 , 38 ). Tumours were also found to express activated forms of Notch1 (ref. 54 ). Therefore, our observation of increased Sox13 and decreased Tcf-1 in IP 3 R KO thymocytes can account for the abnormal thymocyte development observed in our mutants. Full size image The involvement of Ca 2+ signalling and homeostasis in cancer has been well documented, as Ca 2+ signalling regulates numerous pathways involved in proliferation and apoptosis [64] . However, only one other Ca 2+ channel or pump has been directly linked to tumorigenesis in vivo . Mice heterozygous for SERCA2 develop squamous cell carcinomas, which arise as a direct result of SERCA2 haploinsufficiency [65] . The development of leukemia in IP 3 R-TKO mice provides further evidence linking changes in expression and activity of a specific Ca 2+ channel and susceptibility to a specific cancer. Oncogenic transformation of IP 3 R-TKO thymocytes is likely to involve several distinct genetic events. Diminished activity of Tcf-1 has been shown to cause T-cell lymphomas in mice, probably due to deregulation of Lef-1 (ref. 39 ). In agreement with these findings, leukemic thymocytes of IP 3 R-TKO mice have increased levels of Lef-1 expression. Onset of malignancy in IP 3 R-TKO mice occurred at a much earlier age than reported for Tcf-1 −/− mice [39] , suggesting the presence of additional IP 3 R-dependent modifiers, independent of Tcf-1, contributed to disease acceleration. Aberrant activation of Notch1 is the most common oncogenic event observed in T-ALL patients and its expression is tightly regulated in developing thymocytes [48] , [54] . We observed de-repression of several Notch1 transcriptional targets, notably Hes1, in IP 3 R-TKO thymocytes post β-selection. Multiple lines of evidence have demonstrated that Hes1 expression is key to oncogenic transformation of thymocytes. Overexpression of Hes1 in thymocytes leads to a modest ISP developmental block and thymic lymphoma with low penetrance, with lymphomas having ISP and DP signatures [66] . Intriguingly, in light of the overexpression of Id proteins observed in IP 3 R-TKO, Hes1 can also synergize with loss of E protein function to promote oncogenesis. Expression of Hes1 significantly shortens latency of T-cell lymphoma development in Id1 transgenic mice where E protein function is inhibited [66] . Hes1 is also essential for induction of T-ALL by Notch1. Induction of T-ALL on a Hes1-deficient background by overexpressing an oncogenic Notch1 allele results in a significant increase in median survival (25 versus 250 days) [67] . Increased levels of Hes1 in IP 3 R-TKO thymocytes are probably due, at least in part, to decreased expression of Ikaros and Mbd3, the latter a component of the NuRD chromatin-remodelling complex, which represses expression of Notch1 and Hes1 (refs 47 , 48 ). Increased levels of Sox13 and decreased Tcf-1 in IP 3 R-TKO are also likely to contribute to increased expression of Notch targets, including Hes1, as both Tcf-1 −/− and Sox13Tg thymocytes display increased expression of Notch transcriptional targets [37] , [39] , [49] . Although no increases were observed in Notch1 or NICD1 at fetal stages, increases were observed later in hyperplastic thymi and in tumours of IP 3 R-TKO mice. Activating mutations in the Notch1 PEST domain were found to occur spontaneously in tumours of IP 3 R-TKO mice, which suggest a possible tumour suppressing function for IP 3 R and Ca 2+ signalling. Indeed, depletion of ER Ca 2+ stores by treatment with thapsigargin, an inhibitor of the ATP-dependent Ca 2+ pump SERCA, or the knockdown of SERCA impairs Notch receptor maturation in vivo, decreasing the availability of Notch receptors at the cell surface. In this way, ER Ca 2+ homeostasis acts as a major determinant of Notch receptor availability [68] . Inhibition of SERCA also induces a G 0 /G 1 arrest of Notch1 -mutated human T-ALL cell lines. Thus, depletion of ER Ca 2+ stores by the IP 3 R, possibly through pre-TCR signals, might also be expected to impair Notch receptor maturation and decrease availability of Notch receptors at the cell surface. In this manner, IP 3 R signalling may modulate Notch signalling both by transcriptional repression of Notch target genes, as shown in this work, and via regulation of Notch receptor on the cell surface. In apparent contrast to our results, calcineurin, a well-established Ca 2+ -activated phosphatase important for both pre-TCR and TCR signalling, was identified as essential for the survival and maintenance of T-ALL [69] . However, sustained activation of calcineurin in primary T-ALL was found to be independent of pre-TCR and TCR signals. The requirement for Ca 2+ -dependent activation of calcineurin and the role of Ca 2+ signalling in the initiation or maintenance of T-ALL remain to be addressed. Collectively, our results demonstrated that loss of Itpr led to development of T-ALL through multiple collaborative events, including aberrant Sox13 expression, progressive loss of Tcf-1 activity, upregulation of Id proteins, upregulation of Hes1 and, later, activation of Notch signalling. Our data suggest a model in which pre-TCR Ca 2+ signalling through IP 3 R establishes a gene regulatory programme in post β-selected thymocytes that reinforces developmental progression of the αβ T-cell lineage ( Fig. 5 ). In the absence of pre-TCR IP 3 R signalling, T-cell differentiation is arrested at DN4 and ISP stages, and survival and proliferation of ISP thymocytes is compromised. Loss of IP 3 R leads to derepression of the Tcf-1 antagonist Sox13, as well as upregulation of Hes1, at or before the β-selection checkpoint. It is possible, but unlikely, that IP 3 R is required for functions independent of Ca 2+ release. No prior evidence exists that links IP 3 R, a transmembrane ion channel found at the ER and plasma membrane, in directly regulating developmental processes outside of its’ role as a Ca 2+ ion channel. Furthermore, although our results are consistent with a defect in pre-TCR signalling, and Ca 2+ release represents a significant downstream signalling event of the pre-TCR complex, it remains possible that pre-TCR-independent IP 3 R Ca 2+ signalling downstream of other, as yet to be identified, receptors is responsible for the developmental defects observed in mutant thymocytes. We believe this to be unlikely, given the severe disruption in early thymocyte development in LAT Y136F mice in which TCR-mediated Ca 2+ mobilization is specifically impaired [16] . The essential role of TCR-Plcγ1-IP 3 R at later stages of thymocyte development and studies highlighting a role for Ca 2+ in TCR and pre-TCR signalling reinforce this view [2] , [24] , [70] . Of note, the IP 3 R-TKO phenotype we describe is notably less severe than that of homozygous LAT Y136F knock-in mice and raises the possibility that pre-TCR Ca 2+ signalling is not mediated solely through PLCγ1-IP 3 R Ca 2+ release. Additional functions for Ca 2+ in early T-cell development remain to be explored, including the contribution of SOCE-independent Ca 2+ and ion channels to pre-TCR Ca 2+ signalling and development. In summary, our data demonstrate an essential role for IP 3 R Ca 2+ release in pre-TCR signalling and early thymocyte development. Furthermore, this study elucidates a novel role for IP 3 R-mediated signalling in prevention of malignant transformation. Mice The generation of Itpr2 fl and Tie2-Cre has been previously reported [30] , [31] . Rag2 −/− mice were purchased from Taconic. Itpr1 fl/fl and Itpr3 fl/fl mice were generated as described in Supplementary Fig. 1 . All animal experiments were performed according to protocols approved by the UCSD Institutional Animal Care and Use Committee. Flow cytometry and cell sorting Thymocyte suspensions were prepared and filtered through a cell strainer. Antibodies were purchased from eBioscience or BD Pharmingen. Antibodies were directly conjugated to biotin, fluorescein isothiocyanate, phycoerythrin, PE-Cy7, peridinin–chlorophyll–protein complex, PerCP-Cy5.5, allophycoerythrin (APC), or APC-Cy7. The lineage cocktail included antibodies against B220 (RA3-6B3), CD19 (1D3), Ter119 (Ter-119), CD11b/Mac1 (M1/70), Gr1 (8C5), CD11c (HL3), pan-NK/CD49b (DX5), γδ-TCR (GL-3), CD3 (2C11) and CD4 (GK1.5). Additional antibodies used include antibodies against CD8α (53-6.7), TCRβ (H57), c-Kit (2B8), CD25 (PC61.5), CD27 (LG.7F9) and CD44 (IM7). Biotinylated antibodies were stained with a streptavidin-conjugated secondary antibody. Cell sorting was performed on a FACSAria I (BD Biosciences) and flow cytometric analysis was performed on FACSCalibur (BD Biosciences), LSR II (BD Biosciences) and FACSCanto (BD Biosciences). Data were analysed using FlowJo (TreeStar). Western blotting Thymocytes were lysed in SDS loading buffer and fractionated by SDS–PAGE gel electrophoresis, transferred to nitrocellulose membranes and immunoblotted with antibodies to cleaved Notch1 (V1744/NICD1), c-Myc, Ikaros, Mbd3, Tcf-1, Lef1, Sox13, Bcl-x L , E47, HEB, Id2, Id3, p44/42 MAPK (Erk1/2), phopho-p44/42 MAPK (Erk1/2,Thr202/Tyr204), Akt (pan), phospho-Akt (Thr308) and Gapdh. Antibodies against Gapdh were diluted 1:2,000. All others were diluted 1:500. Antibodies were purchased from Cell Signaling Technologies, Sigma-Aldrich and Santa Cruz Biotechnology. Representative uncropped blots are shown in Supplementary Fig. 11 . OP9-DL1 cell culture OP9-DL1 cells were maintained in DMEM supplemented with heat-inactivated fetal bovine serum as previously described [46] . Sca-1 + fetal liver haematopoietic stem and progenitor cells were pre-cultured for 72 h in StemSpan media (Stemcell Technologies) plus human Flt3-L (50 ng ml −1 ), mouse stem cell factor (50 ng ml −1 ) and mouse thrombopoietin (50 ng ml −1 ) to promote hematopoietic stem cell expansion before co-culture with OP9-DL1 cells. For T-cell differentiation assays, thymocyte progenitors or pre-cultured fetal liver stem and progenitor cells were plated onto a monolayer of OP9-DL1 in DMEM plus heat-inactivated fetal bovine serum supplemented with human Flt3-L (5 ng ml −1 ) and mouse interleukin-7 (1 ng ml −1 ). Addition of primary cells to OP9-DL1 was considered Day 0. T-cell development was analysed on Day 12 of co-culture by flow cytometry. Immunohistochemistry Tissues were fixed in 4% paraformaldehyde and embedded in optical coherence tomography. Cryosections (10 μm) were washed with PBS and stained with haematoxylin for 5 min, developed in tap water for 5 min, rinsed twice with deionized water and followed by a 30-s cytoplasmic stain with eosin. Sections were then dehydrated with a gradient of alcohol and xylene, and mounted with Permount. Proliferation and apoptosis assays Animals were injected intraperitonealy with 2 mg bromodeoxyuridine (BrdU; 10 mg ml −1 solution in sterile PBS) and thymocytes were harvested after 4 h. Thymocytes were stained with antibodies and BrdU incorporation was assessed by flow cytometry according to the manufacturer’s instructions (BrdU-APC Kit, BD Pharmingen). Apoptosis was assessed by Annexin-V staining according to the manufacturer’s instructions (Annexin-V FITC Kit, BD Pharmingen). Quantitative RT–PCR RNA was purified from sorted cells using the RNeasy MiniKit (Qiagen) and reverse transcribed to cDNA using SuperScript II Kit (Invitrogen). Real-time PCR was performed with Brilliant II SYBR Green PCR Master Mix (Stratagene) or SSoFast EvaGreen Supermix (Bio-Rad) using gene-specific probes and analysed on MX-Pro (Stratagene) or Roche LightCycler (Roche). Relative transcript abundance was determined by ΔΔCt or ΔCt method after normalization with 18S RNA. All samples were run in duplicate. Error bars represent s.d. Primer sequences are presented in Table 2 . Table 2 Primers used for qRT–PCR analyses. Full size table Gene expression RNA was extracted from sorted neonatal ISP thymocytes (CD4 − CD8 + CD24 hi CD3 − ). RNA from three independent biological replicates were pooled for both wild type and IP 3 R-TKO samples, and submitted to the UCSD Microarray Core Facility. One microarray analysis per pooled sample was performed. All protocols were conducted as described in the Affymetrix GeneChip Expression Analysis Technical Manual. GeneChips used were Affymetrix Mouse Gene1.0ST. Data were analysed using Partek Genomics Suite (Partek). The Database for Annotation, Visualization and Integrated Discovery (DAVID) was used for KEGG pathway analysis. Reported P -values were obtained using a modified Fisher’s exact test. KEGG pathway analyses are shown in Supplementary Tables 1 and 2 . Accession codes : Full gene expression alterations are deposited into the NIH Gene Expression Omnibus ( GSE57997 ). How to cite this article: Ouyang, K. et al. Loss of IP 3 R-dependent Ca 2+ signalling in thymocytes leads to aberrant development and acute lymphoblastic leukemia. Nat. Commun. 5:4814 doi: 10.1038/ncomms5814 (2014).